Extracting net current from an upstream neutral mode in the fractional quantum Hall regime Upstream neutral modes, counter propagating to charge modes and carrying energy without net charge, had been predicted to exist in some of the fractional quantum Hall states and were recently observed via noise measurements. Understanding such modes will assist in identifying the wavefunction of these states, as well as shedding light on the role of Coulomb interactions within edge modes. Here, operating mainly in the ν =2/3 state, we place a quantum dot a few micrometres upstream of an ohmic contact, which serves as a ‘neutral modes source’. We show that the neutral modes heat the input of the dot, causing a net thermo-electric current to flow through it. Heating of the electrons leads to a decay of the neutral mode, manifested in the vanishing of the thermo-electric current at T >110 mK. This set-up provides a straightforward method to investigate upstream neutral modes without turning to the more cumbersome noise measurements. Thirty years after the discovery of the celebrated fractional quantum Hall effect [1] , there are still open questions regarding electronic characteristics in this regime; one of them is the formation and nature of upstream chiral neutral modes. These modes, which carry energy without net charge [2] , [3] , [4] , [5] , [6] , [7] , [8] , [9] , [10] , are at the focus of recent experimental and theoretical studies, and are encouraged by the advent of the search for Majorana quasiparticles [11] , [12] . Certain fractional states, dubbed as hole-conjugate states [13] , [14] , with the most prominent one v =2/3, support reconstructed chiral edge modes, which due to interaction and disorder, give birth to counter propagating neutral modes [2] , [3] , [4] . Among two possible models of the upstream neutral modes: (i) coherent dipole-like excitations, which carry energy; and (ii) classical-like excitations, namely, classical heat waves [15] ; recent results favour the latter one. Being chargeless, the observation of neutral modes presented a challenge. Bid et al. [5] allowed upstream neutral modes, emanating from an ohmic contact, to scatter off a partially pinched quantum point contact (QPC). This has resulted with excess noise but, as expected, with zero net current. In a recent work by Gross et al. [7] , a few new features of these modes were reported: first, that a standard (non-ideal) ohmic contact can detect neutral modes, very much like a QPC; second, injecting charge onto a QPC also excites upstream neutral modes; and third, a simple model of classical heating was found to explain much of the observed data. Moreover, quantum dots (QDs) were used as thermometers to detect temperature increase due to neutral modes [8] , [9] . The results, shown in these precursory works, support energy propagation via upstream chiral neutral modes, and exclude transport of lattice phonons. In this work, we follow a recent proposal, which suggested employing a QD to convert the neutral mode’s energy into a thermo-electric current [10] . We impinged an upstream neutral mode, emanating from the back side of a biased ohmic contact, on the input QPC of a Coulomb blockaded (CB) metallic QD [16] . Conductance peaks exhibited substantial broadening when increasing the bias on the ohmic contact. Furthermore, a net thermo-electric current was generated, due to the temperature gradient across the QD. The results agree with a toy model of a metallic QD having two leads at different temperatures, and the electrons obeying Fermi-Dirac distribution (see more in Supplementary Note S1 and ref. 7 ). Most of the measurements were carried at v =2/3 fractional state, though other filling fractions were also tested. Measurement set-up The sample was fabricated in a GaAs-AlGaAs heterostructure, embedding a two-dimensional electron gas (2DEG) 130 nm below the surface. Schematics of the QD and the measurement set-up are depicted in Fig. 1a ; accompanied by an SEM (scanning electron microscopy) micrograph in Fig. 1b . Because of the relatively short decay length of the neutral modes [5] , the dot, with internal size ~2 × 2 μm 2 , was placed 10 μm upstream of contact N, which served as source for the neutral modes. The current traversing through the dot was measured at contact D, and its root mean square (RMS) value was extracted using a spectrum analyser, thus loosing phase (polarity) information. The sample was cooled to 30 mK in a dilution refrigerator. 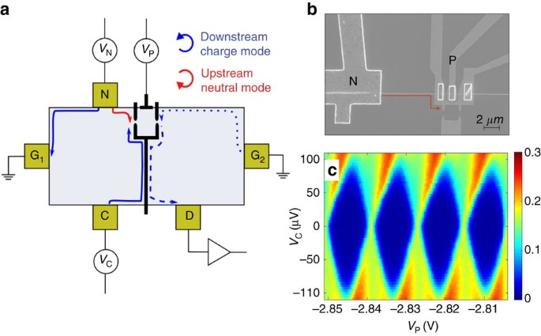Figure 1: Quantum dot scheme. (a) A sketch of the device. Either a charge current injected from contact C (blue) or an upstream neutral current injected from contact N (red) are impinged on the input of the QD. The current at the output of the QD (dashed blue) is measured at contact D through an LC (f0=995 kHz) circuit and a homemade cold amplifier. A constant flow of charged mode fixed at ground potential (contact G2) is impinged on the output side of the dot (blue dotted line). The charge mode emitted from contact N flows directly into the ground (G1, blue) and influences neither the QD nor the experiment. (b) SEM image showing the QD and the ohmic contact used to inject the neutral mode. The upstream neutral current travels a distance of 10 μm along the edge before impinging at the QD (red arrow). All the other ohmic contacts (shown only in panela) are tens of micrometres away from the dot. The QD itself is made out of two QPCs (opening of 650 nm) and a plunger gate (300 nm wide). The lithographic area of the QD is ~2 × 2 μm2. (c) Coulomb diamond characterization of the QD inv=2/3, obtained by measuring the QD’s conductance,, while scanningVPand changingVCin small DC increments. The scale bar is in units of the quantum conductance atv=2/3−G(2e2/3h). Figure 1: Quantum dot scheme. ( a ) A sketch of the device. Either a charge current injected from contact C (blue) or an upstream neutral current injected from contact N (red) are impinged on the input of the QD. The current at the output of the QD (dashed blue) is measured at contact D through an LC ( f 0 =995 kHz) circuit and a homemade cold amplifier. A constant flow of charged mode fixed at ground potential (contact G2) is impinged on the output side of the dot (blue dotted line). The charge mode emitted from contact N flows directly into the ground (G1, blue) and influences neither the QD nor the experiment. ( b ) SEM image showing the QD and the ohmic contact used to inject the neutral mode. The upstream neutral current travels a distance of 10 μm along the edge before impinging at the QD (red arrow). All the other ohmic contacts (shown only in panel a ) are tens of micrometres away from the dot. The QD itself is made out of two QPCs (opening of 650 nm) and a plunger gate (300 nm wide). The lithographic area of the QD is ~2 × 2 μm 2 . ( c ) Coulomb diamond characterization of the QD in v =2/3, obtained by measuring the QD’s conductance, , while scanning V P and changing V C in small DC increments. The scale bar is in units of the quantum conductance at v =2/3− G (2 e 2 /3 h ). Full size image Characterizing of the QD The QD was tuned to the CB regime, having a maximal conductance on resonance. The charging energy was deduced via the ubiquitous non-linear differential conductance (the ‘Coulomb diamond’ in Fig. 1c ) [17] , U c ≈70 μeV and the plunger’s levering factor α P =Δ u /( e Δ V P )=0.005, where Δ u is the dot’s potential. Being relatively large, the QD was metallic, namely δ<<T<<U c , with δ the level spacing and T the electron temperature. Therefore, the dot’s excitation spectrum was practically continuous ( Fig. 1c ), and the width of each conductance peak was expected to be temperature limited [16] , [18] . Heating of the QD’s Input Heating of the QD was monitored by observing the broadening of the conductance peaks in the presence of an upstream neutral mode (red arrow in Fig. 1a ). As V N increased, the conductance peaks broadened (colour scale in Fig. 2a ) while their height hardly changed (see Supplementary Note S2 and Supplementary Figs S1 and S2 ). Two cuts, one at V N =0 and another at V N =200 μV (dashed lines in Fig. 2a ), are shown in Fig. 2b . Employing a two-temperature toy model for the QD, with an input temperature T in and an output temperature of 30 mK, led to T in =125 mK for V N =200 μV. A more complete description of T in ( V N ) is given in Fig. 2c ; it is rather symmetric with respect to V N =0, with a change in slope around V N =150 μV. Such dependence was also observed in previous works [5] , [6] , [7] , [8] . 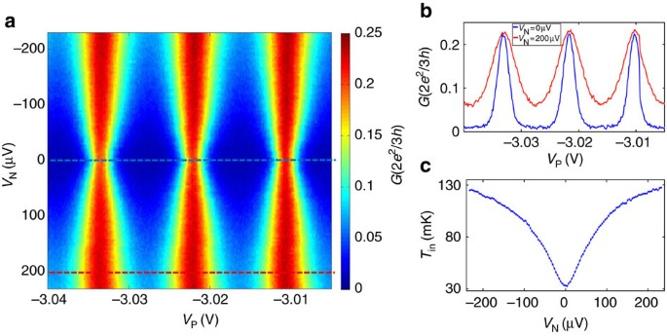Figure 2: Broadening of CB peaks due to neutral mode. (a) 2D plot showing the broadening of three consecutive CB peaks and serving as a proof for the heating caused by the neutral mode. (b) Two cuts of the 2D plot showing CB peaks atVN=0 (blue) andVN=200 μV (red). The dashed lines in panelashow the lines along which the cuts were made. (c) The hot lead’s temperature (Tin) as function ofVN. The values were deduced from the width of the CB peaks using a toy model of a metallic QD with different temperatures at its leads. Figure 2: Broadening of CB peaks due to neutral mode. ( a ) 2D plot showing the broadening of three consecutive CB peaks and serving as a proof for the heating caused by the neutral mode. ( b ) Two cuts of the 2D plot showing CB peaks at V N =0 (blue) and V N =200 μV (red). The dashed lines in panel a show the lines along which the cuts were made. ( c ) The hot lead’s temperature ( T in ) as function of V N . The values were deduced from the width of the CB peaks using a toy model of a metallic QD with different temperatures at its leads. Full size image The above measurements cannot determine whether the dot was heated homogenously or if a temperature gradient was created. In the most naïve approach, current flows in the dot due to the difference between the non-equilibrium energy distributions in both leads [19] . Therefore, when an external bias is applied, electrons will flow from high to low potential with resultant CB peaks ( Fig. 3a ). However, the thermo-electric current I te , driven solely by a temperature gradient across the dot, will strongly depend on the position of the dot’s relevant energy level ( E D ) with respect to the Fermi energy ( ε F ) [20] , [21] . When E D < ε F electrons will flow from the cold to the hot lead, whereas when E D > ε F they will run in the opposite direction ( Fig. 3b ). In Fig. 3c , the blue curve is the measured linear differential conductance, whereas the red curve is the RMS value of thermo-electric current, when V N is AC modulated (amplitude of 10 μV). More information about the sign inversion of I te is presented in Supplementary Fig. S3 and Supplementary Note S3 . This result proves a thermal gradient was formed across the dot due to the upstream neutral mode. 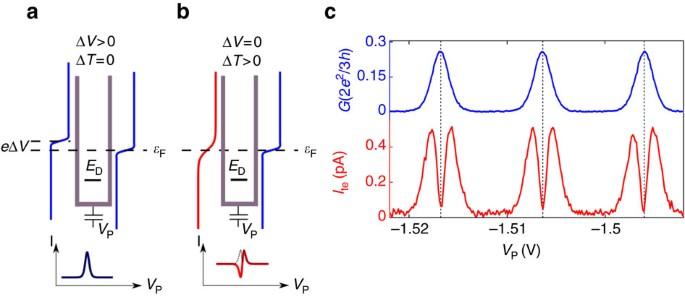Figure 3: Current flow due to either voltage or temperature gradient. An illustration of a quantum dot under electrical or thermal gradient, showing how the current behaves once the QD is near resonance. The energy levels are capacitively coupled to the plunger gate (VP), and for simplicity only one energy level (ED, marked by a full line) is shown. (a) Applying a finite voltage on the left lead will result in current from left to right once the energy level is in the vicinity of the leads’ Fermi energy (εF, marked by dashed line); hence the single peak shown. The blue curve in panelcshows the measured conductance peaks, which fit this picture. (b) Heating up the left lead will result in current from right to left asED<εF, zero current atED=εFand current from left to right whenED>εF. We also show the absolute value of the thermo-electric current (dotted black line) to match our measuring capabilities. The red curve in panelcshows the thermo-electric current due to voltage applied on contact N. The measurement gives a good agreement with the thermal gradient picture. Figure 3: Current flow due to either voltage or temperature gradient. An illustration of a quantum dot under electrical or thermal gradient, showing how the current behaves once the QD is near resonance. The energy levels are capacitively coupled to the plunger gate ( V P ), and for simplicity only one energy level ( E D , marked by a full line) is shown. ( a ) Applying a finite voltage on the left lead will result in current from left to right once the energy level is in the vicinity of the leads’ Fermi energy ( ε F , marked by dashed line); hence the single peak shown. The blue curve in panel c shows the measured conductance peaks, which fit this picture. ( b ) Heating up the left lead will result in current from right to left as E D < ε F , zero current at E D = ε F and current from left to right when E D > ε F . We also show the absolute value of the thermo-electric current (dotted black line) to match our measuring capabilities. The red curve in panel c shows the thermo-electric current due to voltage applied on contact N. The measurement gives a good agreement with the thermal gradient picture. Full size image Thermo-electric current’s dependence on neutral energy Establishing that the heating of the QD is insensitive to the sign of V N ( Fig. 2 ) leads to two possible scenarios: either . This was tested by applying V N = V N,DC + V N,AC cos( ωt ), scanning V N,DC while keeping V N,AC , constant, and measuring the 1st and 2nd harmonics in the current I te . If , then one would expect the 1st harmonic to rise while the 2nd one stays constant while increasing V N,DC . Yet, if I te ∝ | V N |, the 1st harmonic should increase while the 2nd decreases, to eventually disappear once V N,DC > V N,AC . Consequently, the 2nd harmonic is the best criterion to distinguish between the two options. 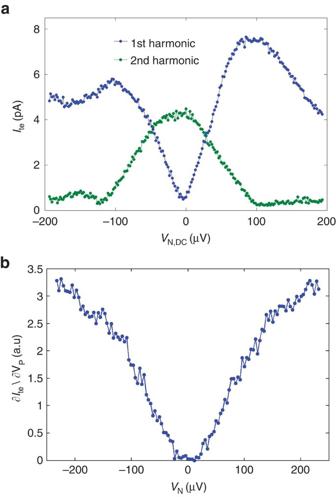Figure 4: Dependence of the resulting thermo-electric signal on the neutral voltage. (a) Change of the thermo-electric current’s first two harmonics when applyingVN=VN,DC+VN,ACcos (ωt) (VN,AC~100 μV). As the 1st harmonic (blue line) increases, the 2nd harmonic (green line) drops. This outcome proves that the thermo-electric currentIteis proportional to |VN|. (b) Amplitude of the thermal transconductance as function of the DC bias onVNwhile keeping a constant AC modulation on the plunger gate. Figure 4a shows the results of such a measurement with f = ω/ 2 π =995 (497.5) kHz when measuring the 1st (2nd) harmonic, V N,AC =100 μV and V N,DC increasing in small increments. The decrease of the 2nd harmonic (green curve), until its diminishing at V N,DC =100 μV= V N,AC , clearly suggests that I te is proportional to | V N | and not to ; as noted in ref. 15 . In addition, the fact that I te followed the ~1 MHz excition on contact N shows that the neutral mode’s response time is 1 μS at most. Figure 4: Dependence of the resulting thermo-electric signal on the neutral voltage. ( a ) Change of the thermo-electric current’s first two harmonics when applying V N = V N,DC + V N,AC cos ( ω t) ( V N,AC ~100 μV). As the 1st harmonic (blue line) increases, the 2nd harmonic (green line) drops. This outcome proves that the thermo-electric current I te is proportional to | V N |. ( b ) Amplitude of the thermal transconductance as function of the DC bias on V N while keeping a constant AC modulation on the plunger gate. Full size image A similar measurement was performed by adding a small AC signal to the plunger gate and varying the DC bias on N. The transconductance was measured at resonance, (where its value is maximal) as function of V N (this is the actual slope of I te at resonance in Fig. 3c (red curve)). The slope in Fig. 4b is a direct representation of I te as function of V N . The slope moderated near V N ~150 μV; attributed to a high enough temperature increase, which may allow two electrons to traverse through the QD—each contributes to an opposite polarity current—leading to the apparent saturation. After establishing a clear indication of heating by the neutral mode, we investigated its dependence on the base temperature. Kane et al. [3] , [4] predicted that the energy carried by the upstream neutral modes decays exponentially with distance, with a characteristic decay length proportional to T −2 , namely, as , with T 0 a characteristic temperature. In the current set-up, raising the lattice temperature (by heating the mixing chamber of the dilution refrigerator, T MC ) should increase the temperature of the output QPC, while lowering the temperature rise at the input QPC. Consequently, the temperature gradient across the QD reduces rapidly, and with it the thermo-electric current should ebb. 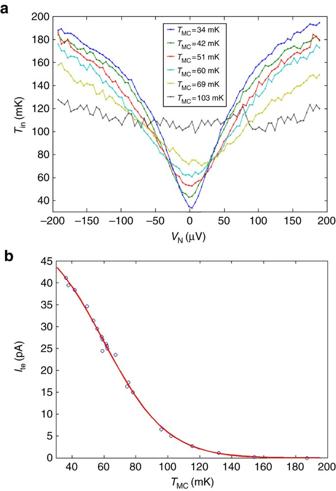Figure 5: Temperature dependence of the neutral modes’ energy. (a) Hot lead’s temperature (Tin) as function of the DC bias on contact N for different base temperatures (34–103 mK). As the temperature increases, the neutral mode’s energy decreases leading to weaker heating of the QD’s input. (b) Thermo-electric current dependence on base temperature, while applying a constant AC signal on contact N. The data is fitted to a quantum dot with a temperature gradient, where. The data (blue circles) is very well described (red line) by our toy model usingα=372 andT0=66 mK. Figure 5a shows T in (deduced in a similar fashion to that described before, see Fig. 2c ) as function of V N at different values of T MC . It is clear that as T MC increases, the temperature rise of the hot input (above T MC ) becomes smaller; without further increase for T MC >100 mK. Via standard noise measurements, we verified that at this base temperature the neutral signal decreased substantially [5] . These results clearly point out a strong decay of the neutral mode with temperature. Figure 5: Temperature dependence of the neutral modes’ energy. ( a ) Hot lead’s temperature ( T in ) as function of the DC bias on contact N for different base temperatures (34–103 mK). As the temperature increases, the neutral mode’s energy decreases leading to weaker heating of the QD’s input. ( b ) Thermo-electric current dependence on base temperature, while applying a constant AC signal on contact N. The data is fitted to a quantum dot with a temperature gradient, where . The data (blue circles) is very well described (red line) by our toy model using α =372 and T 0 =66 mK. Full size image Furthermore, we measured the maximal (as function of V P ) thermo-electric current I te for different values of T MC , while keeping a constant excitation of 300 μV on V N . The data (open circles in Fig. 5b ) was compared with a simulation of I te based on a hot input temperature and a cold output (at T MC ). We found that α =372 mK and T 0 =66 mK lead to an excellent agreement with the data (solid red line in Fig. 5b ); thus supporting the predicted temperature dependence [3] , [4] . Similar measurements were performed at v =3/5, being also a hole-conjugate state, with essentially the same qualitative behaviour [5] . However, no upstream heating had been observed at v =1 and v =2 (ref. 22 ) (as shown in Supplementary Fig. S4 and Supplementary Note S4 ); confirming that the observed heating is due to the presence of upstream neutral modes at certain fractional states. In this work, we demonstrated a new means—exploiting a QD—to transform energy carried by upstream neutral modes into net current; a method that is likely to be simpler than measuring noise. Employing a smaller QD, with a quantized excitation spectrum Δ> T , is expected to provide an experimental gateway to further understanding other properties of the neutral modes [10] . Furthermore, the measurement techniques reported in this work can be used to explore the nature of the neutral modes at the v =5/2 state [5] , [6] , which is suspected to carry with it non-Abelian braiding statistics [23] . Sample fabrication The sample was fabricated in a GaAs-AlGaAs heterostructure, embedding a 2DEG, with areal density 8.8 × 10 10 cm −2 and 4.2 K ‘dark’ mobility 5.8 × 10 6 cm 2 V −1 s −1 , 130 nm below the surface. Schematics of the QD and the measurement set-up are depicted in Fig. 1a ; accompanied by an SEM micrograph in Fig. 1b . The dot, with internal size ~2 × 2 μm 2 , was defined by two split metallic gates (TiAu), serving as QPCs with openings 650 nm wide. A plunger gate, 300 nm wide, controlled the occupation of the dot. Because of the relatively short decay length of the neutral modes [5] , contact N, serving as source for the neutral modes, was placed 10 μm downstream the QD. Contacts C, D, G1 and G2 were placed tens of micrometres away from the dot. The sample was cooled to 30mK in a dilution refrigerator. Measurement technique Biasing contact C raised the chemical potential of the input QPC of the QD, while biasing contact N increased the QPC temperature. In both cases, a net electrical current I traversed the dot. The output drain (D) voltage V D = IR H , with R H , the Hall resistance, was filtered using an LC resonant circuit ( f 0 =995 kHz) and amplified by homemade voltage preamplifier (cooled to 1K) followed by a room temperature amplifier (NF SA-220F5). A commercial spectrum analyser displayed the RMS signal; hence, loosing phase (polarity) information. How to cite this article: Gurman, I. et al. Extracting net current from an upstream neutral mode in the fractional quantum Hall regime. Nat. Commun. 3:1289 doi: 10.1038/ncomms2305 (2012).